Single-molecule chemical reaction reveals molecular reaction kinetics and dynamics Understanding the microscopic elementary process of chemical reactions, especially in condensed phase, is highly desirable for improvement of efficiencies in industrial chemical processes. Here we show an approach to gaining new insights into elementary reactions in condensed phase by combining quantum chemical calculations with a single-molecule analysis. Elementary chemical reactions in liquid-phase, revealed from quantum chemical calculations, are studied by tracking the fluorescence of single dye molecules undergoing a reversible redox process. Statistical analyses of single-molecule trajectories reveal molecular reaction kinetics and dynamics of elementary reactions. The reactivity dynamic fluctuations of single molecules are evidenced and probably arise from either or both of the low-frequency approach of the molecule to the internal surface of the SiO 2 nanosphere or the molecule diffusion-induced memory effect. This new approach could be applied to other chemical reactions in liquid phase to gain more insight into their molecular reaction kinetics and the dynamics of elementary steps. The kinetics of some chemical reactions has been extensively studied with ensemble-averaged methods [1] , [2] . As for the molecular reaction dynamics, only some simple (few atoms) gas-phase elementary reactions have been well studied, based on techniques, such as cross-molecular beams and infrared chemiluminescence [3] , [4] . As for the chemical reactions in condensed phase, much less has been done about the molecular reaction dynamics due to the complexity of traditional methods [5] , [6] . Recent advances in single-molecule fluorescence microscopy have allowed the observations of individual molecules, such as their translational diffusion [7] , [8] , rotational diffusion [9] , spectral fluctuation [10] , conformational motion [11] , the studies of single enzyme or single nanoparticle catalysis [12] , [13] , [14] , [15] , [16] , [17] , and the distinguishing of alternative reaction pathways [18] . Single-molecule measurements can reveal the distributions of molecular static or dynamic properties in inhomogeneous system [19] . These distributions cannot usually be determined by ensemble-averaged methods. Stochastic trajectories from single-molecule experiments contain detailed dynamic information extractable through statistical analysis. For chemical reactions, only the kinetics of some ‘apparent’ non-elementary chemical reactions or process has been studied through single-molecule approach [15] . Of particular interest, however, is the study of molecular reaction kinetics and dynamics via the real-time observation of individual elementary chemical reactions. Here we demonstrate the use of quantum chemical calculations to examine elementary molecular reaction kinetics and dynamics in a homogeneous liquid phase. This is based on a reversible redox process on individual molecules from single-turnover level. Statistical analysis reveals molecular reaction kinetics and dynamics that provide new insight into elementary chemical reactions in condensed phase at single-molecule level. This new information is of great significance for the basic understanding of chemical reactions and their applications. Single-molecule reaction and quantum chemical calculations We found that the fluorescent resorufin (on-state) can be reduced to non-fluorescent dihydroresorufin (off-state) by sodium borohydride (NaBH 4 ) in water under pH 7.3, while the dihydroresorufin can be oxidized easily back to fluorescent resorufin by oxygen ( Fig. 1a ) [20] . This process can be reproduced again and again for many times due to the reversibility of this redox process ( Supplementary Figs 1 and 2 ) [21] , [22] , [23] . 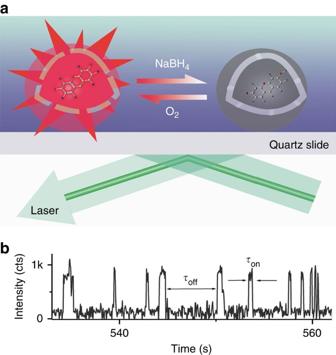Figure 1: Single-turnover detection of single-molecule reaction. (a) Experimental design of single-molecule chemical reaction: a single-resorufin molecule locked in a porous hollow SiO2nanosphere was reduced by NaBH4to non-fluorescent dihydroresorufin, which was then oxidized back to fluorescent resorufin by oxygen. (b) A segment of a typical single-molecule trajectory of fluorescence for the repeated redox process of a single dye molecule. The binning is 50 ms. Figure 1: Single-turnover detection of single-molecule reaction. ( a ) Experimental design of single-molecule chemical reaction: a single-resorufin molecule locked in a porous hollow SiO 2 nanosphere was reduced by NaBH 4 to non-fluorescent dihydroresorufin, which was then oxidized back to fluorescent resorufin by oxygen. ( b ) A segment of a typical single-molecule trajectory of fluorescence for the repeated redox process of a single dye molecule. The binning is 50 ms. Full size image The above repetitive fluorescence on-off phenomenon is the basis for observation of real-time single-molecule reaction by detecting the fluorescence of the same single dye molecule repeatedly at single-reaction single-turnover level. To monitor the individual chemical reactions in situ , first, porous hollow SiO 2 nanospheres [24] with inner diameter about 210 nm ( Supplementary Fig. 3 ) were filled with diluted resorufin aqueous solution to form SiO 2 /Dye complex (no. of resorufin molecules ≤1 for each nanosphere, for details see Supplementary Methods and Discussion ), then immobilized on quartz surface and flowed the substrate solution over (containing both reductant NaBH 4 and oxidant O 2 ; Fig. 1a ). Using an inverted total internal reflection fluorescence microscope with down to 50 ms integration time and 532 nm laser excitation, we recorded movies of stochastic fluorescence bursts at some localized spots. A typical time trajectory of fluorescence intensity from these spots contains stochastic on-off digital signal that spans the entire movie (up to 1 h, Fig. 1b and Supplementary Fig. 2 ). The digital nature of the trajectory and the consistent height of the on-level indicate that each fluorescence burst comes from a single-resorufin molecule [15] . We attributed the single-resorufin fluorescence bursts to a single-turnover of the reversible redox reaction as shown in Fig. 1 . Each time when the resorufin is formed by the oxidation of the only dihydroresorufin molecule in a SiO 2 nanosphere, a sudden increase in intensity is seen in the fluorescence trajectory. In contrast, each time when the only resorufin molecule in this nanosphere is reduced to nonfluorescent dihydroresorufin by NaBH 4 , a sudden decrease in intensity is seen. This, each on-off cycle, corresponds to a single turnover of the reversible redox reaction. All the turnovers on each trajectory are due to the repeated redox process of the same single dye molecule. This is different from that observed on single-molecule single-nanoparticle catalysis [15] , [25] , in which each burst comes from a new or different product molecule. Many observations support our conclusion. (1) No digital fluorescence bursts are observed in the absence of SiO 2 /Dye complex. (2) Only short lifetime (with average lifetime ~1 min) blinking and photobleaching are observed in the absence of NaBH 4 , O 2 or both ( Supplementary Fig. 4 ). (3) The fluorescence bursts are not photoinduced ( Supplementary Fig. 5 ) [15] . As shown in Fig. 1b , there are two waiting times in these single-molecule fluorescence trajectories. Resolving them enables us to probe the kinetic mechanism of this chemical reaction from single-molecule level in two parts separately: τ on (approximate waiting time needed for the reduction of resorufin) and τ off (approximate waiting time needed for the oxidation of dihydroresorufin back to resorufin). Their individual values are stochastic, but their statistical properties, such as average values and distribution, are well defined by the underlying reaction kinetics. Statistically [15] , in this case, ‹τ on › −1 and ‹τ off › −1 , where ‹› denotes averaging, represent the time-averaged single redox reaction rates of reduction and oxidation processes, respectively. When averaged over the turnover trajectories from many individual redox molecules, ‹ τ on › −1 and ‹ τ off › −1 , should be expectedly dependent on reductant or oxidant concentrations, respectively, and exhibit saturation kinetics [14] . In order to tell the on- and off-process precisely, we need to know the detailed reduction mechanism and the fluorescence states of all the stable intermediates. For that goal, the NaBH 4 reduction mechanism was studied in detail to find the most feasible reaction pathways and stable intermediates by quantum chemical calculation ( Supplementary Methods and Discussion ). NaBH 4 has been extensively used as reducing agent for organic chemistry [26] , [27] , [28] , [29] . Previous work [20] , [29] , [30] has shown that the reducing process of resorufin by NaBH 4 should follow the attacking of BH 4 − to the carbonyl group to form IM1 first ( Fig. 2a ) and finally, the hydrolysis of IM2 to product dihydroresorufin. After investigating several possible mechanisms ( Supplementary Fig. 6 ), the optimal one with smallest energy barrier was determined, as shown in Fig. 2a . 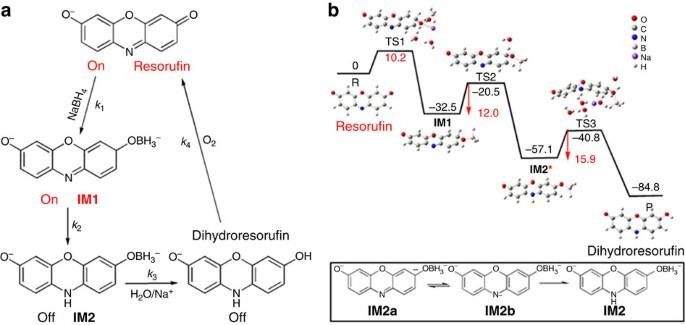Figure 2: The mechanism of single-molecule chemical redox reaction based on quantum chemical calculation. (a) Schematic diagram of the mechanism for the redox process of single dye (resorufin) molecules. The fluorescence state (on or off) of the dye is indicated at each reaction step. (b) The energy profile for resorufin reduction by NaBH4(kcal mol−1). Inset:IM2*represents there is one fast charge rearrangement process fromIM2atoIM2b(bottom inset), and then spontaneous protonation process toIM2. Figure 2b is the corresponding energy profile for this reduction pathway. Here it was found that Na + cation and water molecule have participated in the first transition state collectively via the nucleophilic addition of BH 4 − to the carbonyl group in resorufin, which occurs easily due to a very small activation energy. Obviously the process from substrate to IM1 is an elementary step. It was confirmed here that the proton on the C atom in the carbonyl group could be taken off easily by water from IM1 to form IM2a , with a small energy barrier of 12.0 kcal mol −1 . The C atom in sp 3 hybridization in IM2a tends to turn into sp 2 hybridization to form another resonance structure with stable phenyl ring in IM2b . This was followed by the spontaneous fast protonation process on the N atom (inset in Fig. 2b ), that is, the intermediate IM2b and then IM2 . So the rate constant k 2 approximately represents reactivity of the slow elementary step from IM1 to IM2a . The hydrolysis process of IM2 , an elementary-reaction step, occurred via a larger activation energy to form the reduction product dihydroresorufin, where Na + cation and water also play an important role. In other words, the hydrolysis process ( k 3 ) is the rate-determining step in the whole reduction process, which is consistent with the long τ off observed in the following single-molecule experiments. For the oxidation process, dihydroresorufin is known to be easily oxidized by oxygen back to the initial substrate resorufin [20] . This molecule will go to the next redox cycle again and again. The quantum chemical calculations have also been carried out to predict the properties for ground state (S 0 ) and singlet excited state (S 1 ) of the intermediates found in the reduction process. The results show the intermediate IM1 can still emit strong fluorescence due to the intact planar π system, and intermediate IM2 shows turned-off fluorescence due to the distorting non-planar Λ-type geometry (see Supplementary Table 1 ). As this calculation can reliably predict the fluorescence states of the initial substrate (resorufin) and the final product dihydroresorufin, the predictions for the two intermediates ( IM1 and IM2 ) seem plausible. Figure 2: The mechanism of single-molecule chemical redox reaction based on quantum chemical calculation. ( a ) Schematic diagram of the mechanism for the redox process of single dye (resorufin) molecules. The fluorescence state (on or off) of the dye is indicated at each reaction step. ( b ) The energy profile for resorufin reduction by NaBH 4 (kcal mol −1 ). Inset: IM2* represents there is one fast charge rearrangement process from IM2a to IM2b (bottom inset), and then spontaneous protonation process to IM2 . Full size image Molecular reaction kinetics and dynamics of elementary reactions Based on the above information, we can tell that the τ on process includes the steps shown in Fig. 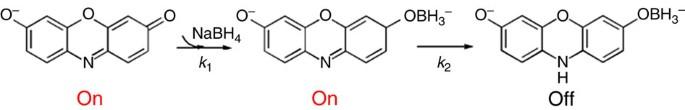Figure 3: The mechanism of theτonprocess. . 3 : Figure 3: The mechanism of the τ on process. . Full size image The ‘on’ represents either resorufin or IM1 . Following a single-molecule kinetic analysis ( Supplementary Methods and Discussion ) [31] , we get the probability density function of τ on , f on (τ) as The reciprocal of the first moment of f on (τ), ‹ τ on › −1 , represents the reduction rate of a dye molecule: Equation (2) connects τ on , a stochastic single-molecule quantity, with conventional kinetic parameters and predicts the saturation kinetics of ‹ τ on › −1 . Fitting the molecule-averaged data of ‹ τ on › −1 at different [NaBH 4 ], shown in Fig. 4a , gives k 1 =522±90 mM −1 s −1 and k 2 =4.93±0.05 s −1 , both values here reflecting averaged properties of many dye molecules. 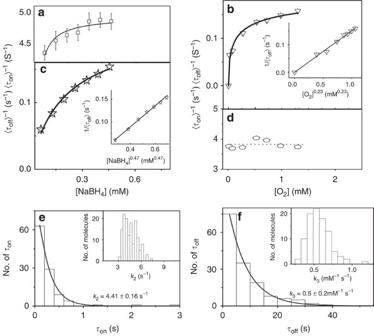Figure 4: Molecular reaction kinetics. Reductant and oxidant concentration dependence of ‹τon›−1(a,d) and ‹τoff›−1(b,c). Each data point is an average from about 80 trajectories. Solid lines are fits from Equations (2), (4) and (5). Errors are s.d. Experiments for (a,c) are in water solution with 1.3 mM O2, for (b,d) are in water solution with 0.26 mM NaBH4. Insets: the linear dependence of turnover rate on [O2]0.23(c) and [NaBH4]0.47(b). (e)The on-time distribution derived from redox process of a single dye molecule with 0.45 mM NaBH4and 1.3 mM O2(k2being the rate-limiting step forτon). Solid line is the single exponential fit withk2=4.41±0.16 s−1. Inset is the distribution ofk2derived from about 90 dye molecules in the same sample. (f) The off-time distribution derived from redox process of a single dye molecule with 0.26 mM NaBH4and 1.3 mM O2(k3being the rate-limiting step forτoff). Solid line is the single exponential fit withk3=0.5±0.2 mM−1s−1. Inset is the distribution ofk3derived from about 90 dye molecules in the same sample. Note thatk2andk3are time averaged over entire trajectories. Figure 4: Molecular reaction kinetics. Reductant and oxidant concentration dependence of ‹ τ on › −1 ( a , d ) and ‹ τ off › −1 ( b , c ). Each data point is an average from about 80 trajectories. Solid lines are fits from Equations (2), (4) and (5). Errors are s.d. Experiments for ( a , c ) are in water solution with 1.3 mM O 2 , for ( b , d ) are in water solution with 0.26 mM NaBH 4 . Insets: the linear dependence of turnover rate on [O 2 ] 0.23 ( c ) and [NaBH 4 ] 0.47 ( b ). ( e )The on-time distribution derived from redox process of a single dye molecule with 0.45 mM NaBH 4 and 1.3 mM O 2 ( k 2 being the rate-limiting step for τ on ). Solid line is the single exponential fit with k 2 =4.41±0.16 s −1 . Inset is the distribution of k 2 derived from about 90 dye molecules in the same sample. ( f ) The off-time distribution derived from redox process of a single dye molecule with 0.26 mM NaBH 4 and 1.3 mM O 2 ( k 3 being the rate-limiting step for τ off ). Solid line is the single exponential fit with k 3 =0.5±0.2 mM −1 s −1 . Inset is the distribution of k 3 derived from about 90 dye molecules in the same sample. Note that k 2 and k 3 are time averaged over entire trajectories. Full size image The above model also predicts that the τ on process has nothing to do with [O 2 ]. In the single-molecule experiments with a wide range of different [O 2 ] and the same [NaBH 4 ], ‹ τ on › −1 roughly showed no change, as shown in Fig. 4d . For the τ off process, it contains the steps shown in Fig. 5 . 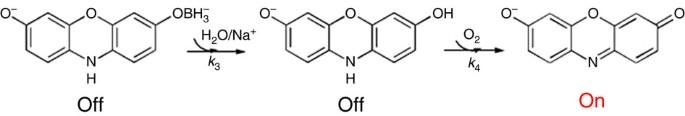Figure 5: The mechanism of theτoffprocess. . Figure 5: The mechanism of the τ off process. . Full size image It clearly shows the τ off is not a pure oxidation process of dihydroresorufin. It contains the hydrolysis process of IM2 and the oxidation process of dihydroresorufin by O 2 . As the quantum chemical calculation ( Fig. 2 ) shows the Na + cation, which mainly comes from NaBH 4 , participates in the hydrolysis process of IM2 , the ‹ τ off › −1 should depend on both [NaBH 4 ] and [O 2 ]. Following a similar single-molecule kinetic analysis, we get the probability density function of τ off ( Supplementary Methods and Discussion ): When we vary the concentration of NaBH 4 with constant [O 2 ], Equation (3) can be simplified as: with . Then Fitting the molecule-averaged data of ‹ τ off › −1 at different [NaBH 4 ] with fixed O 2 concentration, as shown in Fig. 4c , gives k 3 =1.1±0.1 mM −1 s −1 and k 4 0 =0.23±0.02 s −1 . As the O 2 concentration is about 1.3 mM in this case, then k 4 is about 0.22 mM −1/2 s −1 . Similarly, when we vary the O 2 concentration with constant [NaBH 4 ], the probability density function of τ off , f off (τ) is with . and Here, the rate constant k 3 contains water contribution as its concentration is very high and keeps constant during the whole reaction process. Fitting the molecule-averaged data at different [O 2 ], shown in Fig. 4b , gives k 3 0 =0.21±0.02 s −1 and k 4 =0.4±0.1 mM −1/2 s −1 . Based on [NaBH 4 ]=0.26 mM, k 3 is estimated to be about 0.81 mM −1 s −1 , which reflects the rate of the hydrolyzation of intermediate IM2 . Compared with k 1 and k 2 for τ on , the much smaller k 3 and k 4 indicate the τ off is a much slower process than τ on . That is why ‹ τ off › observed here is much longer than ‹ τ on ›. As shown above, two independent experiments that had varying reductant and oxidant concentrations were used to determine k 3 and k 4 , respectively. Values obtained for k 3 and k 4 are within the same order of magnitude and approximately consistent within error range. The differences in values of k 3 and k 4 are about 26 and 45%, respectively. The big differences probably come from the estimation error of NaBH 4 concentration due to its slow hydrolysis process. The reduction process of resorufin by NaBH 4 was studied precisely based on elementary steps discriminated from quantum chemical calculation. This provided detailed kinetic information for each elementary step, helping us to understand elementary chemical reactions more deeply. This has not been shown in previous reports. Obviously the fine discrimination and the kinetic study of elementary chemical reactions usually cannot be done with traditional ensemble-averaged methods. The new knowledge obtained in this approach, such as the rate constants for some rate-limiting elementary steps, is of great significance for the optimization of chemical reactions. On the other hand, from the above we can see the apparent net reaction is: The total turnover rate r total = k app [NaBH 4 ] n [O 2 ] k , where n , k are the real reaction orders with respect to NaBH 4 and O 2 , respectively. For single dye molecule-based reaction occurred in individual SiO 2 hollow nanospheres, , in the concentration range of NaBH 4 and O 2 used in the present work, , so . As the τ off process is related to [NaBH 4 ] according to Equation (4), when [O 2 ] is fixed, by fitting the data shown in the inset of Fig. 4c , and n with respect to NaBH 4 were obtained to be about 0.225±0.004 mM −0.47 s −1 and 0.47±0.01, respectively. Similarly for O 2 , when [NaBH 4 ] is fixed, , as shown by the fit in the inset of Fig. 4b , and k were obtained to be 0.15±0.01 mM −0.23 s −1 and 0.23±0.01, respectively. Obviously in this special case the real reaction orders ( n =0.47, k =0.23) with respect to NaBH 4 and O 2 are different from the stoichiometric coefficients (1 and 1/2). This phenomenon has been extensively observed before based on ensemble-averaged methods [32] . It is interesting to see that the ratio between the reaction order n and k is 2, the same as the ratio between the stoichiometric coefficients. Furthermore, based on the obtained n and k , k app is obtained to be about 0.25 mM −0.7 s −1 . The disclosure of the real reaction orders and apparent rate constant for single-molecule chemical reactions above exemplifies a new power of single-molecule method in revealing the molecular reaction dynamics. The probability density function of τ on , as shown in Equation (1), is the convolution of two exponentials ( k 1 [NaBH 4 ] and k 2 ) [33] . In this case, k 1 =522±90 mM −1 s −1 and k 2 =4.93±0.05 s −1 . The much larger k 1 0 (= k 1 [NaBH 4 ]) than k 2 makes the convolution in τ on invisible even at the lowest concentration of NaBH 4 (0.065 mM), at which we can only see the monotonic decay, as is the case observed before for single nanoparticle catalysis [15] . On the other hand, when [NaBH 4 ]→∞, . It predicts that the waiting time ( τ on ) distribution for each single molecule should be a single exponential when the reductant concentration is high enough. As an example shown in Fig. 4e at high reductant concentration, from the decay constant we obtained the rate constant of k 2 for this single molecule to be about 4.41±0.16 s −1 . To see the static heterogeneity of this type of molecule, we obtained the values of k 2 for many individual molecules. From the distribution (insert in Fig. 4e with ‹ k 2 ›=4.62±0.89 s −1 ) we can see the difference is very big among these individual molecules, although they are all exactly the same in chemical composition and physical structure. Similarly, the probability density function of τ off (Equation (3)) is the convolution of two exponentials ( k 3 [NaBH 4 ] and k 4 [O 2 ] 1/2 ). We checked the τ off distributions for all the trajectories at different [NaBH 4 ] or [O 2 ] concentrations; some distributions from single-molecule trajectories (about 1%) show the obvious convolution of two exponentials ( Supplementary Fig. 7 ). However, from these distributions we cannot get precise values for the rate constants from the double-exponential fitting ( Supplementary Methods and Discussion ). On the other hand, for Equation (3b), when[O 2 ]→ ∞ , . Thus, we can get the value of k 3 from for each individual molecule from single exponential distribution of waiting time ( τ off ) when the oxidant concentration is high enough. Indeed, as shown in Fig. 4f , we obtained the rate constant of k 3 for a single molecule to be about 0.5±0.2 mM −1 s −1 . The values of k 3 for many individual molecules (insert in Fig. 4f ) also show big static heterogeneity of this type of molecule with ‹ k 3 ›=0.54±0.15 mM −1 s −1 . These static heterogeneities could be partially attributed to the heterogeneous microenvironments around each molecule. The different microenvironments probably could be attributed to the static heterogeneity of individual SiO 2 nanospheres, such as different sizes, porosities and surface patterns in nanospheres. The reactivity dynamic fluctuations of single molecules From each single-turnover trajectory, we further determined the time dependence of the turnover rates (the number of off-on cycles per second; Fig. 6a ). Large temporal variations were observed, indicating dynamic reactivity fluctuations of individual dye molecules, consistent with the revelations from the Poisson indicator ( P ) [34] , which is related to the second moment of f ( t ) ( Supplementary Figs 8 and 9 ). The reactivity fluctuations could be related to reaction rate changes in the τ on or τ off process. To assess the contribution of τ on and τ off processes to the reactivity fluctuations, we extracted the sequence of individual τ on and τ off from each turnover trajectory, and then calculated their autocorrelation functions C τ ( m )=‹Δ τ (0)Δτ( m )›/‹Δ τ 2 › (refs 14 , 15 , 35 ). Here, τ is either τ on or τ off , m is the turnover index number in the sequence and Δτ( m )= τ ( m )−‹ τ ›, the delay time. In the presence of reactivity fluctuations, C τ ( m )>0 shows a decay behaviour with the decay time constant being the fluctuation correlation time [14] , [35] . 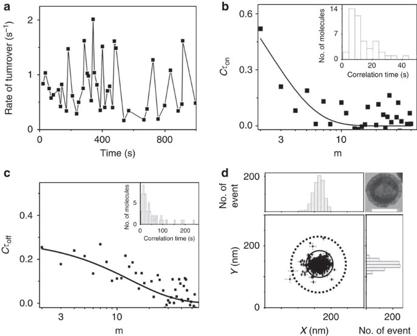Figure 6: Single-molecule reaction dynamics. (a) Trajectory of turnover rate (s−1) for a single dye molecule at 0.45 mM NaBH4and 1.3 mM O2. Data points are calculated every five turnovers. (b,c) Autocorrelation functions ofτonandτoffderived from the same trajectory as that in a. Solid lines are the exponential fits with decay constants ofmon=2.3±0.7 andmoff=13.3±5.5 turnovers. Insets: Histograms of fluctuation correlation times forτon(k2) andτoff(k3). (d) Mapping of Brownian motion of a single dye molecule inside a hollow SiO2nanosphere with optical super-resolution imaging. The dotted circle indicates the inner cavity of the nanosphere; the solid one indicates the centre area of the cavity. Top left: the distribution of the dye inx-direction; Bottom right: the distribution of the dye iny-direction; Top right: a typical transmission electron microscopy image of a hollow SiO2nanosphere, the scale bar, 200 nm. Figure 6: Single-molecule reaction dynamics. ( a ) Trajectory of turnover rate (s −1 ) for a single dye molecule at 0.45 mM NaBH 4 and 1.3 mM O 2 . Data points are calculated every five turnovers. ( b , c ) Autocorrelation functions of τ on and τ off derived from the same trajectory as that in a. Solid lines are the exponential fits with decay constants of m on =2.3±0.7 and m off =13.3±5.5 turnovers. Insets: Histograms of fluctuation correlation times for τ on ( k 2 ) and τ off ( k 3 ). ( d ) Mapping of Brownian motion of a single dye molecule inside a hollow SiO 2 nanosphere with optical super-resolution imaging. The dotted circle indicates the inner cavity of the nanosphere; the solid one indicates the centre area of the cavity. Top left: the distribution of the dye in x -direction; Bottom right: the distribution of the dye in y -direction; Top right: a typical transmission electron microscopy image of a hollow SiO 2 nanosphere, the scale bar, 200 nm. Full size image For a dye molecule in a hollow SiO 2 nanosphere at saturating reductant (0.45 mM of NaBH 4 ) or oxidant (1.3 mM of O 2 ) concentrations, both and show exponential decay, indicating both reduction and hydrolysis rates fluctuate or a memory effect [14] . For instance, as shown in Fig. 6b, c , the decay constants are m on =2.3±0.7 and m off =13.3±5.5 turnovers obtained from two different trajectories with [NaBH 4 ] and [O 2 ] saturated, respectively. These two trajectories were from NaBH 4 - and O 2 -titration experiments, respectively, as shown above. With average turnover time of 9.3 and 6.2 s for these two turnover trajectories, the fluctuation correlation times for τ on and τ off related to the delay process are ~21.4 and ~72.5 s, respectively. These two correlation times reflect the fluctuation or delay timescales of k 2 and k 3 , which are rate-limiting in τ on and τ off processes at saturating reductant and oxidant concentrations. These two steps also are the key elementary steps for the reduction process of dye by NaBH 4 and could never be resolved and studied separately by any traditional method. The insets in Fig. 6b,c show the histograms of fluctuation correlation time of τ on ( k 2 ) and τ off ( k 3 ) processes from many individual dye molecules; their broad distributions indicate that the reactivity of these resorufin molecules fluctuates in very different timescales. To further confirm the existence of dynamic disorder or memory effect, we presented a statistical analysis of two-dimensional conditional probability distributions for a pair of adjacent on-times and off-times, as shown in Supplementary Fig. 10 , no diagonal features could be seen clearly, indicating that the two-dimensional histograms of waiting times are not sensitive to the dynamic disorder or memory effect [14] , similar to that previously observed for single nanoparticle catalysis [15] . Interestingly, here a long timescale from seconds to tens of seconds has been observed from the on-time and off-time autocorrelation functions. The long autocorrelation time indicates a slow fluctuation of the microenvironment. Obviously, solvent rearrangements and vibrational or rotational motion of the dye molecule occur on a tremendously faster timescale than the observed decays. So what kind of fluctuations of the microenvironment around the dye molecules occur on such a slow timescale? The first reason probably could be due to the low-frequency approaching or contact of single dye molecule to the internal surface of SiO 2 nanosphere. Each time when the free dye molecule approaches to the Si or O atoms on the internal surface of SiO 2 nanosphere, its reactivity with reductant or oxidant probably will be affected due to the asymmetric microenvironment (one side is solid wall, the other side is liquid) [36] , [37] . In order to confirm above analysis, we applied a Monte-Carlo simulation to mimic the Brownian motion of a single dye molecule confined in the nanosphere ( Supplementary Methods and Discussion ). The Monte-Carlo time with unit mcs (Monte-Carlo step) and the times of the contact between dye molecule and internal surface of the hollow nanosphere were recorded ( Supplementary Table 2 ). It shows, when the sphere diameter is increased from 20 to 200 (10 times), the average waiting time for a contact between the dye molecule and the internal surface of the nanosphere is increased from 43 to 6,510 mcs (more than 150 times). According to previous results for particle Brownian motion [38] , [39] , the long waiting time of 6,510 mcs could approximately correspond to a real-time scale of up to second. So, the low-frequency approaching of dye molecule to the inner surface of SiO 2 nanosphere probably contributes in part to the slow fluctuation of microenvironment around the single dye molecule. Another possible reason for the slow fluctuation of microenvironment was single-molecule diffusion-induced memory effect, which was observed unexpectedly in the following single-molecule tracking analysis (see more discussions there). Both the τ off and τ on processes probably depend on the same fluctuations mentioned above, but maybe in different ways, which then leads to different decays of τ off and τ on . To get more clues about reactivity dynamic fluctuation of single dye molecules, we used the fitting of the emission point spread function [40] , [41] , the basis for optical super-resolution imaging methods [23] , [42] , [43] , to ‘track’ the movement of single dye molecules in SiO 2 nanospheres. In this way, we can map the location variation of a free single dye molecule in situ inside the cavity of a hollow SiO 2 nanosphere during the repeated redox process ( Supplementary Methods and Discussion ; Supplementary Figs 11 and 12 ). Centre locations of single dye molecule at different time were obtained from many τ on periods in one fluorescence trajectory with better than 10 nm precision. As shown in Fig. 6d , all the centres of the same dye molecule in the on-state from different τ on appear in a circle with diameter about 150 nm, which is close to the averaged inner diameter of hollow SiO 2 nanospheres used here (top right: transmission electron microscopy image). To get more information from the Brownian motion of single dye molecule inside the SiO 2 nanosphere, the position of dye molecule on each frame of τ on was obtained and analysed deeply. According to the scheme shown in Fig. 7a , we calculated two sequences of distances from each trajectory: D 1 { a 1 a 2 , a 2 a 3 ,… a n− 1 a n , b 1 b 2 , b 2 b 3 ,.. b n− 1 b n ,…} sequence for the molecule on two adjacent frames in the same τ on , such as between a i (or b i , c i … ) and a i+ 1 (or b i+ 1 , c i+ 1 … ) ( i =1, 2… n ); Dk { a n b 1 , b n c 1 ,… d n e 1 …} sequence for the molecule on two frames exactly separated by a τ off , such as between a n (or b n , c n … ) and b 1 (or c 1 , d 1 …). It was found that the averaged Dk (36±6 nm), the distance for the molecule before/after multiple steps diffusion, is much longer than the averaged D 1 (26±4 nm), the distance for the molecule on two adjacent frames or the diffusion step-size, indicating a divergent diffusion pattern of the molecule. Furthermore, we calculated the autocorrelation coefficients for these two sets of distances ( D 1 and Dk ), respectively. Interestingly, the D 1 sequence shows strong positive autocorrelation with coefficient of ρ =0.425. While the Dk sequence shows no autocorrelation ( ρ =−0.05). These data unambiguously show a dynamic disorder or a memory effect related to the diffusion of dye molecule, indicating a short diffusion-step tends to be followed by another short step, and a long step tends to be followed by another long step. The molecule diffusion-induced memory effect has been realized to be the basis of molecular communication [44] , [45] . In it, the messages can be conveyed via the variation in the concentration of molecules in the small-scale medium. However, due to the delay of the variation of concentration of molecules, the dynamic disorder or memory effect appears during the molecule diffusion process [44] . 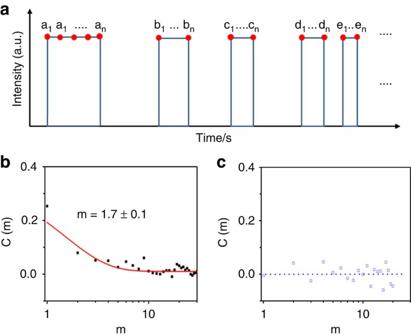Figure 7: Diffusion-induced memory effect of single dye molecule in the hollow SiO2nanosphere. (a) The scheme to show how the distance sequences (D1andDk) were calculated fromτonon a fluorescence trajectory.D1:{a1a2,a2a3,…an−1an,b1b2,b2b3,..bn−1bn,…} for the molecule on two adjacent frames in the sameτon;Dk:{anb1,bnc1,…dne1…} for the molecule on two frames exactly separated by aτoff(nis the total number of frames in oneτon, and the value should be different for differentτon). (b,c) The autocorrelation functions of the distance sequences (D1(b) andDk(c)). The solid line inbis the exponential fit with decay constant ofm=1.7. Themis the index number in sequence. Figure 7: Diffusion-induced memory effect of single dye molecule in the hollow SiO 2 nanosphere. ( a ) The scheme to show how the distance sequences ( D 1 and Dk ) were calculated from τ on on a fluorescence trajectory. D 1 :{ a 1 a 2 , a 2 a 3 ,… a n− 1 a n , b 1 b 2 , b 2 b 3 ,.. b n− 1 b n ,…} for the molecule on two adjacent frames in the same τ on ; Dk :{ a n b 1 , b n c 1 ,… d n e 1 …} for the molecule on two frames exactly separated by a τ off ( n is the total number of frames in one τ on , and the value should be different for different τ on ). ( b , c ) The autocorrelation functions of the distance sequences ( D 1 ( b ) and Dk ( c )). The solid line in b is the exponential fit with decay constant of m =1.7. The m is the index number in sequence. Full size image To evaluate the timescale of this diffusion-induced memory effect in this case, we further calculated the autocorrelation function for the data sets ( D 1 and Dk ). Interesting, as an example shown in Fig. 7b , the decay constant for the successive diffusion steps ( D 1 sequence) is m =1.7, corresponding to the autocorrelation time of about 0.1 s, further confirming a dynamic disorder or a memory effect ( Supplementary Fig. 13a ) [14] . While as shown in Fig. 7c , distances ( Dk sequence) for the points separated by multiple ( ⩾ 2) frames show no autocorrelation or memory effect ( Supplementary Fig. 13b ). These facts are consistent with previous observation due to a molecule diffusion-based memory effect [44] . From multiple individual molecules, we found the averaged diffusion-induced autocorrelation time is about 0.5 s. The slow timescale observed here is approximately in the range of that observed from τ on and τ off autocorrelation shown in Fig. 6 . So the diffusion-induced dynamic fluctuation observed here may also contribute in part to the slow dynamic fluctuation of the microenvironment or the reactivity of single dye molecules. Here we examined the kinetics and dynamics of three tandem homogeneous elementary chemical reactions in real time from single-molecule level at single-turnover resolution. This study exemplifies a new powerful tool of quantum chemical calculation-based single-molecule approach in revealing new insight of elementary molecular reaction kinetics and dynamics. By this approach, the molecular reaction kinetics, dynamics and the reactivity dynamic fluctuation of a complex chemical process in a homogeneous liquid phase were studied thoroughly from an elementary-reaction level. In principle, this new approach may be applicable for some other chemical reactions in liquid phase to get more insight about their molecular reaction kinetics and dynamics for elementary steps. Hollow SiO 2 nanoparticle synthesis and characterization The hollow SiO 2 nanoparticles were synthesized in two steps. Briefly, solid SiO 2 spheres were made first, and then etched to hollow mesoporous silica nanospheres with wormhole-like shell. These SiO 2 nanospheres are hollow and porous in structure with inner diameters about 210 nm averagely. Single-molecule chemical reaction experiments Single-molecule fluorescence measurements were performed on a homebuilt prism-type total internal reflection fluorescence microscope based on an Olympus IX71 inverted microscope. A continuous wave circularly polarized 532 nm laser beam (CrystaLaser, GCL-025-L-0.5%) of 4–5 mW was focused onto an area of ~80 × 80 μm 2 on the sample to directly excite the fluorescence of resorufin. The fluorescence of resorufin was collected by a × 60 NA1.2 water-immersion objective (UPLSAPO60XW, Olympus), filtered by two filters (HQ550LP, HQ580m60), and projected onto a camera (Andor iXon EMCCD, DU-897U-CS0-#BV), which is controlled by an Andor IQ software. All optical filters are from Chroma Technology. The movies are analysed using a home-written IDL program, which extracts the fluorescence intensity trajectories from localized fluorescence spots individually across the entire movie. The intensity of each bright spot in an image is obtained by integrating the signal counts over an area of ~1 × 1 μm 2 . A flow cell, 100 μm (height) × 2 cm (length) × 5 mm (width), formed by double-sided tapes sandwiched between a quartz slide (Technical Glass or Finkenbeiner) and a borosilicate coverslip (Gold Seal), was used to hold aqueous sample solutions for single-molecule fluorescence measurements. A volume of 100 μl of 1 nM colloidal hollow SiO 2 or SiO 2 /Dye complex solution was spin-coated onto quartz slide, and then rinsed several times with MilliQ water to remove unbound nanoparticles. On the quartz slide, two holes were drilled to connect to polyethylene tubing and a syringe pump for continuous solution flow at 10 μl min −1 . Quantum chemical calculations Density functional theory (DFT) method at M062X/6-31+G* level has been carried out to calculate the stationary point with frequency computations. The total energy has been corrected by higher accurate second-order Møller-Plesset perturbation theory (MP2) level using 6-311++G** basis set with solvation effect. The solvent effect in water was employed by using SMD solvent method, which can be more accurate for charged species than other solvent models. All the reactant, intermediates and product have been confirmed to be the minimum with no imaginary frequencies, and each transition state had only one imaginary frequency. How to cite this article: Zhang, Y. et al . Single-molecule chemical reaction reveals molecular reaction kinetics and dynamics. Nat. Commun. 5:4238 doi: 10.1038/ncomms5238 (2014).